HDL-transferred microRNA-223 regulates ICAM-1 expression in endothelial cells High-density lipoproteins (HDL) have many biological functions, including reducing endothelial activation and adhesion molecule expression. We recently reported that HDL transport and deliver functional microRNAs (miRNA). Here we show that HDL suppresses expression of intercellular adhesion molecule 1 (ICAM-1) through the transfer of miR-223 to endothelial cells. After incubation of endothelial cells with HDL, mature miR-223 levels are significantly increased in endothelial cells and decreased on HDL. However, miR-223 is not transcribed in endothelial cells and is not increased in cells treated with HDL from miR-223 −/− mice. HDL inhibit ICAM-1 protein levels, but not in cells pretreated with miR-223 inhibitors. ICAM-1 is a direct target of HDL-transferred miR-223 and this is the first example of an extracellular miRNA regulating gene expression in cells where it is not transcribed. Collectively, we demonstrate that HDL’s anti-inflammatory properties are conferred, in part, through HDL-miR-223 delivery and translational repression of ICAM-1 in endothelial cells. Numerous population studies have established that plasma high-density lipoprotein (HDL) cholesterol levels inversely correlate with cardiovascular risk [1] , [2] , [3] , [4] . The most extensively studied cardio-protective function of HDL particles relate to their participation in the reverse cholesterol transport pathway [5] . Studies from this and other laboratories have shown that HDL also repress inflammatory gene expression in cytokine-activated endothelial cells and other cell types [6] , [7] , [8] , [9] . Nevertheless, the underlying mechanisms conferring their cardio-protective effects are poorly understood largely because HDL are heterogeneous and consist of several structurally and functionally distinct subpopulations of particles [3] , [10] , [11] , [12] , [13] . We have recently reported that HDL also transport specific microRNAs (miRNAs) [14] , [15] . miRNAs are small non-coding RNAs that post-transcriptionally regulate gene expression through translational inhibition and mRNA destability [16] . They have proven to be powerful regulators of many biological processes, including cellular growth, metabolism, physiology and response to stress [17] , [18] . They are also stably found in both cells and extracellular compartments, such as plasma, and regulate gene expression [15] , [19] . Circulating miRNAs are potential novel class of biomarkers for cardiovascular disease and have the capacity to act as bioactive signalling molecules [17] , [20] . Altered extracellular miRNA profiles have been observed in inflammation, cardiovascular diseases, atherosclerosis, diabetes, obesity and ageing [19] , [21] . miRNAs are transcribed as primary transcripts (pri-miRNA) and further processed into precursor (pre-miRNA) hairpins in the nucleus [22] . Upon nuclear export, miRNAs are cleaved to their mature forms [22] . Recently, it has been shown that mature miRNAs are likely involved in intercellular communication, a process by which miRNAs are transferred between cells by lipid-based carriers, including exosomes, microvesicles and lipoproteins. As such, mature miRNAs are able to regulate gene expression in cells in a novel form of endocrine-like cell-to-cell communication [14] , [15] , [23] , [24] , [25] , [26] , [27] , [28] . miR-223 is a miRNA that is of particular interest in cardiovascular disease as its levels are significantly increased in HDL from humans and mice with hypercholesterolaemia [14] . Moreover, miR-223 is one of the most abundant miRNAs in monocytes and macrophages and a key regulator of inflammation [29] . miR-223-null ( miR-223 −/− ) mice have a significantly increased number of circulating neutrophils and enhanced systemic inflammation following a lipopolysaccharide challenge [29] . In this study, we demonstrate that the anti-inflammatory properties of HDL are conferred, in part, by the transfer of miR-223 to recipient endothelial cells where it suppresses adhesion molecule expression. Within this study, we extensively characterized the gene (mRNA) and miRNA signatures of human coronary artery endothelial cells (HCAEC) following incubation with HDL, which transport miRNAs including miR-223 or the individual constituents of HDL. Studies were also carried out with reconstituted HDL consisting of 1-palmitoyl-2-linoleoyl phosphatidylcholine (PLPC) and apoA-I (rHDL), lipid-free apolipoprotein A-I (apoA-I) and PLPC small unilamellar vesicles (SUV). Results indicate that native HDL particles and their individual lipid and apolipoprotein constituents differentially alter the expression of numerous genes and the levels of several miRNAs in HCAEC. Moreover, we found that HDL transfer of miR-223 to endothelial cells, where miR-223 is not transcribed or processed, contributes to the mechanisms by which HDL inhibit inflammation in HCAEC. HDL constituents control gene expression in HCAEC HDL have previously been reported to alter gene expression in multiple cell types; however, it is unclear whether it is the lipid or apolipoprotein constituents, with apoA-I being the most abundant HDL apolipoprotein, that contribute to this gene regulation [5] , [12] , [30] . To characterize the endothelial cell response to intact native HDL particles, as well as to their lipid and apolipoprotein constituents, non-activated HCAEC were incubated for 16 h with native human HDL, rHDL, lipid-free apoA-I or SUV. Results from SDS–PAGE analyses indicate that the apoA-I preparations were >95% pure ( Supplementary Fig. 1A ). The rHDL preparations had a final PLPC/apoA-I molar ratio of 80:1 and consisted of three subpopulations of particles with 8.7, 9.8 and 11.8 nm diameters ( Supplementary Fig. 1B ). 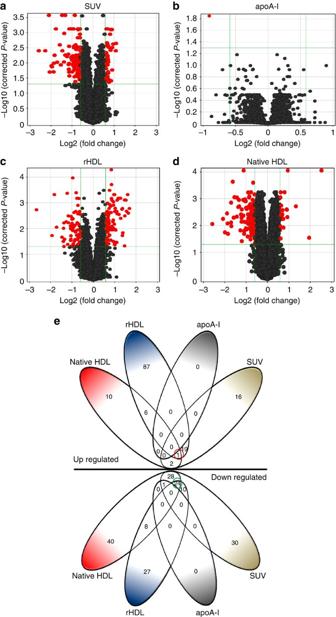Figure 1: HDL and its components distinctly alter gene expression in human endothelial cells. (a) HCAEC were incubated at 37 °C for 16 h with SUV (final PLPC concentration 3 mmol l−1), (b) lipid-free apoA-I (final concentration 1 mg ml−1), (c) rHDL (final apoA-I concentration 1 mg ml−1) or (d) native human HDL (final total protein concentration 1 mg ml−1). Volcano plots of significant and differential HCAEC gene expression changes are shown for five separate experiments (≥1.5-fold, Benjamini–Hochberg-correctedP<0.05). Red dots indicate genes with ≥1.5-fold change (Log2 fold change) andP<0.05 (−Log10 correctedP-value). (e) Venn diagram of overlapping gene changes. Green circle (24 genes) and red circle (1 gene) identify common HCAEC genes that were respectively downregulated or upregulated by SUV, rHDL and native HDL. The plasma concentration of human HDL constituents is presented in Supplementary Table 1 . These preparations consisted of multiple subpopulations of particles ranging from ~7.0 to 10.0 nm in diameter ( Supplementary Fig. 1C ). Changes in gene (mRNA) expression were analysed by whole-genome gene arrays. Significant and differential gene changes were observed in HCAEC treated with SUV (124 in total; 31 up; 93 down), lipid-free apoA-I (1 down), rHDL (182 in total; 113 up; 69 down) and native human HDL (120 in total; 19 up; 101 down) (Benjamini–Hochberg-corrected P <0.05; ≥1.5-fold; Fig. 1a–d red circles, Supplementary Data 1 ). Each HDL constituent, except lipid-free apoA-I, significantly altered the expression of a diverse set of genes, many of which are associated with inflammation ( Supplementary Data 1 ). Strikingly, a group of shared genes were similarly altered (24 downregulated, green circle; 1 upregulated, red circle) by SUV, rHDL and native HDL ( Fig. 1e ). As the common feature of SUV, rHDL and native HDL is their ability to accept unesterified cholesterol from cell membranes, these genes are likely altered in response to cholesterol efflux, and therefore, were classified as the ‘cholesterol efflux responsive gene set’ ( Fig. 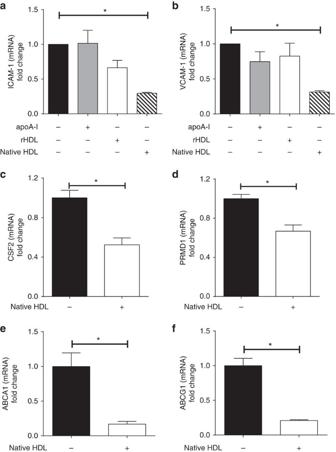Figure 2: HDL inhibits genes associated with inflammation and cholesterol efflux in endothelial cells. ICAM-1 (a) and VCAM-1 (b) mRNA expression in HCAEC incubated with lipid-free apoA-I, rHDL or native HDL as described in the legend toFig. 1. CSF2 (c), PRMD1 (d), ABCA1 (e) and ABCG1 (f) mRNA levels in HCAEC incubated with native HDL, as quantified by real-time PCR. All data are presented as mean±s.e.m. (N≥4). Mann–Whitney nonparametric test was used to compare two independent groups with a sample size >3. When data were paired and samples size was >3, Wilcoxon-matched-pairs tests were used. *P<0.05. 1e green and red circles, Supplementary Table 2 ). 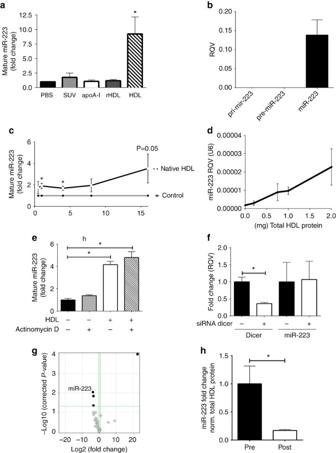Figure 3: HDL transfers miR-223 to human endothelial cells. (a) HCAEC were incubated with native HDL, lipid-free apolipoprotein A-I (apoA-I), discoidal reconstituted HDL (rHDL) or SUV as described in the legend toFig. 1. Intracellular levels of mature miR-223 were quantified by real-time PCR using individual TaqMan miRNA assays. RQV (normalized to U6) are reported as fold change (N=5). (b) Primary miR-223 (pri-mir-223, TaqMan Assays), precursor miR-223 (pre-miR-223, SYBR green assays), and mature miR-223 (TaqMan assays) levels in HCAEC. RQV normalized to peptidylprolyl isomerase A (PPIA) (N=4). (c) Intracellular miR-223 levels in HCAEC after incubation with native HDL (final protein concentration 1 mg ml−1) for 30 min, 1, 4, 8 or 16 h, normalized to U6 and reported as fold change (N=5–8). (d) Intracellular levels of miR-223 levels in HCAEC incubated with increasing doses of HDL treatments for 24 h. Results are normalized to U6 and reported as RQV (N=3). (e) Intracellular miR-223 levels in HCAEC pre-incubated with actinomycin D (5 μg ml−1, 8 h) followed by native HDL incubation for 24 h, as quantified by real-time PCR, normalized to PPIA and reported as fold change. (N=3). (f) Intracellular levels of Dicer1 and miR-223 in HCAEC transfected with 100 nM siRNA against Dicer1, as quantified by real-time PCR. Results are normalized to PPIA and reported as fold change. (N=4). (g) miRNA profiling of HDL before (pre) and after (post) incubation with HCAEC. Real-time PCR-based TaqMan Low-Density miRNA arrays. Values are presented as a volcano plot of significant and differential HDL-associated miRNA changes (≥1.5-fold,P<0.05). (h) Validation of miR-223 levels in HDL pre/post incubation with HCAEC, as quantified by individual TaqMan miRNA assays. (N=4). All data are presented as mean+s.e.m. Unpaired two-tailed Student’st-test was used when comparing two groups with a sample size ≥3. Mann–Whitney nonparametric test was used to compare two independent groups with a sample size >3. When data were paired and samples size was >3, Wilcoxon matched-pairs tests were used. To compare three or more unmatched groups, one-way ANOVA and the Tukey’s multiple comparisons post-test was used. *P<0.05. Ingenuity Pathway Analyses identified 19 significantly downregulated pathways and 1 upregulated pathway associated with the cholesterol efflux responsive gene set, with the interferon signalling pathway being the most significantly altered pathway ( Supplementary Table 3 ). 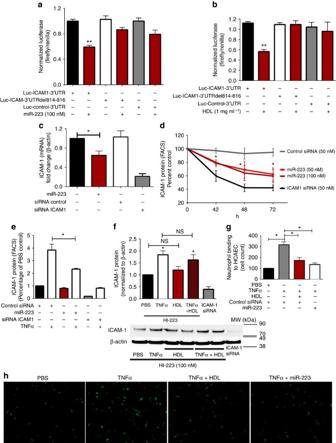Figure 4: miR-223 directly target ICAM-1 in HCAEC. (a) Normalized (Firefly/Renilla) luciferase activity in HEK 293 cells dual transfected for 48 h with miR-223 and luciferase gene reporters containing the full-length ICAM-1–3′ UTR, a three-nucleotide (814–816) deletion in the predicted miR-223 target site or a control-3′ UTR.N=3–9 (b) Normalized (Firefly/Renilla) luciferase activity in HCAEC transfected with luciferase gene reporters containing the full-length ICAM-1–3′ UTR, a three-nucleotide (814–816) deletion or control-3′ UTR for 24 h and incubated for a further 24 h with or without native HDL.N=3–18 (c) ICAM-1 mRNA levels in HCAEC transfected (48 h) with miR-223, control siRNA or targeting pool siRNA ICAM-1.N=5–7 (d) ICAM-1 protein levels 24, 48 and 72 after HCAEC were transfected with miR-223, ICAM-1 siRNA or control siRNA, as quantified by flow cytometry.N=4 (e) ICAM-1 protein levels in HCAEC 72 h after miR-223, control siRNA or ICAM-1 siRNA transfection followed by ±TNF-α (2 ng ml−1) for 5 h.N=3–4 (f) ICAM-1 protein levels in HCAEC transfected with miR-223 hairpin inhibitor, or ICAM-1 siRNA for 24 h followed by native HDL or PBS incubations (16 h) and ±TNF-α for a further 5 h.N=3–6 (a–f) All data are represented as mean±s.e.m. (g,h) Neutrophil-binding assays in activated HCAEC as described in theSupplementary InformationN=4. The numbers of adherent neutrophils are presented with values representing the mean+s.e.m. Unpaired two-tailed Student’st-test was used when comparing two groups with a sample size ≤3. Mann–Whitney nonparametric test was used to compare two independent groups with a sample size >3. When data were paired and samples size was >3, Wilcoxon matched-pairs tests were used. To compare three or more unmatched groups, one-way ANOVA and Tukey’s multiple comparisons post-test were used. *P<0.05, **P<0.01. 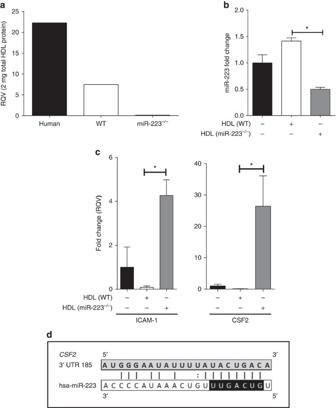Figure 5: HDL repression of inflammatory gene expression in HCAEC. (a) RQV of miR-223 levels in HDL isolated from human and mouse plasma by fast-protein liquid chromatography (FPLC). Mouse plasma was pooled from sixmiR-223−/−mice and 12 WT mice for FPLC separation. (b,c) HCAEC were incubated with pooled native HDL (final total protein concentration 1 mg ml−1) from WT ormiR-223−/−mice for 24 h. (b) miR-223 levels were quantified by real-time PCR and normalized to U6 levels (RQV=2−(miR-223 Ct—U6 Ct)). (N=2–3). (c) ICAM-1 and CSF2 mRNA levels were quantified by real-time PCR and normalized to peptidylprolyl isomerase A (PPIA) levels (RQV). (N=2–3). (d) Predicted miR-223 target site within the 3′ untranslated region (3′ UTR) of the CSF2 (mRNA) gene. Most importantly, each HDL constituent significantly altered distinct canonical pathways: native HDL treatment altered 26 pathways ( Supplementary Table 4 ), rHDL treatment altered 19 pathways ( Supplementary Table 5 ) and SUV treatment altered 25 pathways ( Supplementary Table 6 ). The most altered pathway by native HDL was the clathrin-mediated endocytosis signalling pathway ( Supplementary Table 4 ). Other signalling pathways that were altered by incubation with HDL included the inflammatory nuclear factor-kappaB (NF-κB) signalling pathway ( Supplementary Table 4 ). Within the NF-κB pathway, interleukin 33 ( IL33 , −1.75-fold, Benjamini–Hochberg-corrected P <0.05), phosphatidylinositol-4-phosphate 3-kinase C2 domain-containing beta polypeptide ( PIK3C2B , −1.5-fold, Benjamini–Hochberg corrected P <0.01) and tumor necrosis factor, alpha-induced protein 3 ( TNFAIP3 , −1.88-fold, Benjamini–Hochberg corrected P <0.01) were all significantly decreased at the mRNA level ( Supplementary Table 7 ). Figure 1: HDL and its components distinctly alter gene expression in human endothelial cells. ( a ) HCAEC were incubated at 37 °C for 16 h with SUV (final PLPC concentration 3 mmol l −1 ), ( b ) lipid-free apoA-I (final concentration 1 mg ml −1 ), ( c ) rHDL (final apoA-I concentration 1 mg ml −1 ) or ( d ) native human HDL (final total protein concentration 1 mg ml −1 ). Volcano plots of significant and differential HCAEC gene expression changes are shown for five separate experiments (≥1.5-fold, Benjamini–Hochberg-corrected P <0.05). Red dots indicate genes with ≥1.5-fold change (Log2 fold change) and P <0.05 (−Log10 corrected P -value). ( e ) Venn diagram of overlapping gene changes. Green circle (24 genes) and red circle (1 gene) identify common HCAEC genes that were respectively downregulated or upregulated by SUV, rHDL and native HDL. Full size image Native HDL gene regulation is distinct from its components To determine which genes in HCAEC are regulated specifically by native HDL, the genes that were altered only by apoA-I, rHDL and SUV treatments were excluded from the analysis. Using this approach, we identified 49 unique genes that were altered in HCAEC by native HDL treatments alone ( Supplementary Table 7 ). It is well established that increased vascular cell adhesion molecule 1 (VCAM-1) and intercellular adhesion molecule 1 (ICAM-1) expression in response to endothelial activation is mediated through the transcription factor NF-κB [31] , [32] . We have previously reported that HDL inhibit cytokine-induced ICAM-1 and VCAM-1 expression in activated endothelial cells through the NF-κB pathway [7] , [33] , [34] . To determine whether HDL suppress inflammatory gene expression as a homoeostatic mechanism, whole-genome gene arrays were used with RNA from non-activated HCAEC. We found that ICAM-1 mRNA levels were significantly decreased by incubation with both HDL (−1.44-fold, Benjamini–Hochberg-corrected P =0.01, not shown on Supplementary Data 1 , which only includes genes significantly altered ≥1.5-fold) and SUV (−1.54-fold, Benjamini–Hochberg-corrected P <0.05, Supplementary Data 1 ) after 16 h. Moreover, VCAM-1 mRNA levels were also found to be significantly decreased by HDL (−2.49-fold, Benjamini–Hochberg-corrected P <0.01, Supplementary Data 1 ) and SUV (−1.85-fold, Benjamini–Hochberg-corrected P <0.05, Supplementary Data 1 ) treatments. Real-time PCRs were used to further confirm that incubation of non-activated HCAEC with native HDL resulted in significant loss of endothelial cell ICAM-1 ( Fig. 2a ) and VCAM-1 ( Fig. 2b ) mRNA levels. Lipid-free apoA-I, by contrast, failed to significantly reduce adhesion molecule expression in non-activated HCAEC ( Supplementary Data 1 , Fig. 2a,b ). Figure 2: HDL inhibits genes associated with inflammation and cholesterol efflux in endothelial cells. ICAM-1 ( a ) and VCAM-1 ( b ) mRNA expression in HCAEC incubated with lipid-free apoA-I, rHDL or native HDL as described in the legend to Fig. 1 . CSF2 ( c ), PRMD1 ( d ), ABCA1 ( e ) and ABCG1 ( f ) mRNA levels in HCAEC incubated with native HDL, as quantified by real-time PCR. All data are presented as mean±s.e.m. ( N ≥4). Mann–Whitney nonparametric test was used to compare two independent groups with a sample size >3. When data were paired and samples size was >3, Wilcoxon-matched-pairs tests were used. * P <0.05. Full size image Granulocyte-macrophage colony-stimulating factor (GM-CSF), product of the CSF2 gene, is a major pro-inflammatory cytokine that is secreted from endothelial cells, fibroblasts and inflammatory cells [35] , [36] , [37] . Most interestingly, we found that native HDL treatment significantly decreased CSF2 mRNA levels in HCAEC ( Fig. 2c ). In addition to CSF2, other inflammatory genes were also found to be suppressed by HDL treatments, including chemokine (C–C motif) ligand 20 ( CCL20 ) and chemokine (C–X–C motif) ligand 1 ( CXCL1 ) ( Supplementary Data 1 ). CXCL1 is another endothelial cytokine involved in both inflammation and angiogenesis [38] . Moreover, incubations with native HDL also decreased the mRNA levels of PR domain zinc finger protein 1 ( PRDM1 or BLIMP-1 ) in non-activated endothelial cells ( Fig. 2d ). PRDM1 is a key transcriptional repressor of beta-interferon expression and plays a pivotal role in inflammation, haematopoietic stem cell differentiation and beta-lymphocyte maturation into antibody-producing cells [39] . Strikingly, we found that ATP-binding cassette transporter G1 ( ABCG1 ) mRNA levels were significantly decreased in HCAEC treated with SUV (−2-fold, Benjamini–Hochberg-corrected P <0.01), rHDL (−2.4-fold, Benjamini–Hochberg-corrected P <0.01) and native HDL (−1.7-fold, Benjamini–Hochberg-corrected P <0.01) ( Supplementary Data 1 ). Endothelial cell ATP-binding cassette transporter A1 ( ABCA1 ) mRNA levels were also significantly decreased by rHDL (−1.95-fold, Benjamini–Hochberg-corrected P =0.0001, Supplementary Data 1 ), SUV (−1.4-fold, Benjamini–Hochberg-corrected P <0.01) and native HDL (−1.4-fold, Benjamini-Hochberg–Hochberg- P <0.01) treatments (not shown on Supplementary Data 1 , which only includes genes significantly altered ≥1.5-fold). Results for HDL treatments were confirmed by real-time PCR ( Fig. 2e–f ). HDL alters endothelial cell miRNA levels To determine whether HDL, SUV, lipid-free apoA-I or rHDL differentially alter miRNA levels in endothelial cells, real-time PCR-based TaqMan miRNA arrays were used to profile HCAEC miRNA levels before and after treatments. HDL, SUV, lipid-free apoA-I and rHDL all distinctly altered endothelial cell miRNAs ( Supplementary Fig. 2 , Table 1 ). Significant differential miRNA changes were observed in endothelial cells treated with SUV (1 down), lipid-free apoA-I (18 in total; 15 down; 3 up), rHDL (5 in total; 1 down; 4 up) and native HDL (3 in total; 1 down; 2 up) (unpaired t -test P <0.05; ≥1.5-absolute fold; Table 1 , Supplementary Fig. 2A–D ). Strikingly, only native human HDL treatments were found to significantly increase intracellular mature miR-223 levels in HCAEC (16.5-fold, unpaired t -test P <0.001, Table 1 ). This was confirmed by real-time PCR in replicate studies ( Fig. 3a ). PBS incubation was used as a control. Table 1 Significant differential endothelial cell miRNA expression in response to HDL components. Full size table Figure 3: HDL transfers miR-223 to human endothelial cells. ( a ) HCAEC were incubated with native HDL, lipid-free apolipoprotein A-I (apoA-I), discoidal reconstituted HDL (rHDL) or SUV as described in the legend to Fig. 1 . Intracellular levels of mature miR-223 were quantified by real-time PCR using individual TaqMan miRNA assays. RQV (normalized to U6) are reported as fold change ( N =5). ( b ) Primary miR-223 (pri-mir-223, TaqMan Assays), precursor miR-223 (pre-miR-223, SYBR green assays), and mature miR-223 (TaqMan assays) levels in HCAEC. RQV normalized to peptidylprolyl isomerase A (PPIA) ( N =4). ( c ) Intracellular miR-223 levels in HCAEC after incubation with native HDL (final protein concentration 1 mg ml −1 ) for 30 min, 1, 4, 8 or 16 h, normalized to U6 and reported as fold change ( N =5–8). ( d ) Intracellular levels of miR-223 levels in HCAEC incubated with increasing doses of HDL treatments for 24 h. Results are normalized to U6 and reported as RQV ( N =3). ( e ) Intracellular miR-223 levels in HCAEC pre-incubated with actinomycin D (5 μg ml −1 , 8 h) followed by native HDL incubation for 24 h, as quantified by real-time PCR, normalized to PPIA and reported as fold change. ( N =3). ( f ) Intracellular levels of Dicer1 and miR-223 in HCAEC transfected with 100 nM siRNA against Dicer1, as quantified by real-time PCR. Results are normalized to PPIA and reported as fold change. ( N =4). ( g ) miRNA profiling of HDL before (pre) and after (post) incubation with HCAEC. Real-time PCR-based TaqMan Low-Density miRNA arrays. Values are presented as a volcano plot of significant and differential HDL-associated miRNA changes (≥1.5-fold, P <0.05). ( h ) Validation of miR-223 levels in HDL pre/post incubation with HCAEC, as quantified by individual TaqMan miRNA assays. ( N =4). All data are presented as mean+s.e.m. Unpaired two-tailed Student’s t -test was used when comparing two groups with a sample size ≥3. Mann–Whitney nonparametric test was used to compare two independent groups with a sample size >3. When data were paired and samples size was >3, Wilcoxon matched-pairs tests were used. To compare three or more unmatched groups, one-way ANOVA and the Tukey’s multiple comparisons post-test was used. * P <0.05. Full size image In HCAEC, SUV treatments were found to only alter one miRNA in either direction, miR-296-3p (−1.75-fold). Although lipid-free apoA-I treatments were found to only downregulate a single gene at the mRNA level ( Fig. 1b ), these treatments resulted in the significant increase and decrease of 3 and 15 miRNAs, respectively, including miR-100 (−1.76-fold), miR-17* (miR-17-3p, -3.97-fold) and miR-548p (4.18-fold). rHDL treatments were found to increase four miRNAs, including miR-496 (2.91-fold), and decrease 1 miRNA, miR-943 (−2.61-fold, Table 1 ). Although multiple miRNAs were significantly altered in these incubations, we failed to identify miRNAs that changed in the same direction (either upregulated or downregulated) in incubations of HCAEC with any two of the following: HDL, rHDL, lipid-free apoA-I or SUV. To determine whether there are possible shared miRNAs that just missed our statistical cutoff of P values <0.05 and fold changes >1.5, we loosened the stringency for filtering. First, we compared miRNAs that were statistically different for each condition (unpaired t -test P <0.1). After grouping miRNAs by directional trend (up and down), we generated Venn diagrams to identify overlapping miRNA changes ( Supplementary Fig. 3A,B ). This strategy failed to find any overlap with the downregulated miRNAs ( Supplementary Fig. 3B ); however, in the upregulated set, two miRNAs were found to be commonly regulated by rHDL and SUV, one miRNA by apoA-I and SUV, one miRNA by HDL and rHDL, one miRNA by apoA-I and rHDL and 1 miRNA by HDL and apoA-I. We also found one miRNA to be upregulated by apoA-I, SUV and rHDL ( Supplementary Fig. 3A ). Secondly, we filtered miRNAs that were found to be altered >1.5-absolute fold change, independent of P values and statistical comparisons. Although less stringent than our previous analyses, this strategy identified numerous miRNA commonly up- or downregulated by HDL, rHDL, lipid-free apoA-I and SUV ( Supplementary Fig. 4A,B ). We found 86 miRNAs commonly upregulated (>1.5-fold) by at least two conditions (>1.5-fold, Supplementary Fig. 4A ), 15 of which were upregulated by all apoA-I containing particles (rHDL, lipid-free apoA-I and native HDL). Moreover, we identified one miRNA, miR-548L, that was upregulated in all four conditions. In the miRNAs that were found to be downregulated >−1.5-fold, we identified 53 miRNAs commonly downregulated by at least two conditions ( Supplementary Fig. 4B ). Moreover, we found six miRNAs that were downregulated by all apoA-I containing particles (rHDL, lipid-free apoA-I and native HDL) ( Supplementary Fig. 4B ). Mature miR-223 is transferred from HDL to endothelial cells To determine whether the intracellular increase in miR-223 levels was due to induced transcription and processing or exogenous uptake, we designed a series of in vitro studies to assess HDL-mediated endothelial cell effects. To distinguish between these two possibilities, miR-223 transcription and processing was assessed in HCAEC after HDL treatments. Most importantly, no evidence was found to suggest that miR-223 is transcribed in endothelial cells, as primary mir-223 (pri-mir-223) and precursor miR-223 (pre-miR-223) transcripts were undetectable by real-time PCR ( Fig. 3b ). Furthermore, the observed increase in intracellular miR-223 levels was apparent after 30 min of incubation with native HDL, statistically significant at 1 h ( Fig. 3c ). These data suggest that the observed increases in cellular miR-223 levels are likely due to HDL transfer of miR-223, and not a consequence of increased transcription. This is consistent with the findings that mature miR-223 levels increased in a concentration-dependent manner in the HCAEC incubated with increasing HDL concentrations ( Fig. 3d ). To determine whether the absence of miR-223 transcription was specific to HCAEC, basal levels of pri-mir-223 and mature miR-223 were also quantified in human umbilical vascular endothelial cells (HUVEC) ( Supplementary Fig. 5A ). Similarly to HCAEC, there was no evidence of miR-223 transcription in HUVEC, as pri-mir-223 transcripts were undetectable by real-time PCR. Mature miR-223 levels in HUVEC were found to be significantly lower than in HCAEC (unpaired two-tailed Student’s t -test P =0.0002, Supplementary Fig. 5A ). Furthermore, native HDL treatments increased intracellular mature miR-223 levels by 16.1-fold in the HUVEC (Mann–Whitney nonparametric test P <0.05, Supplementary Fig. 5B ). To further rule out the possibility of HDL-induced miR-223 transcription in HCAEC, cells were incubated with native HDL and Actinomycin D, a chemical inhibitor of transcription. HDL-induced miR-223 changes were found to be transcription-independent, as HDL incubations in the presence or absence of Actinomycin D both significantly increased miR-223 levels 4.2- and 4.8-fold, respectively ( Fig. 3e ). These results further support the possibility that the increase in endothelial cell miR-223 levels reflects the transfer from HDL, rather than increased miR-223 transcription. To establish that this observation is unique to miR-223, we quantified miR-29a, a miRNA present in HCAEC, and found that neither HDL, nor Actinomycin D and HDL treatments resulted in an increase in intracellular miR-29a levels ( Supplementary Fig. 6A ). To demonstrate that Actinomycin D was successful in inhibiting transcription in these conditions, ICAM-1 and VCAM-1 mRNA levels were quantified in the presence or absence of Actinomycin D with or without HDL ( Supplementary Fig. 6B,C ), and we found that these mRNAs were highly sensitive to the loss of transcription in these cells. To demonstrate that miR-223 is not likely processed in HCAEC, we used siRNAs to knockdown Dicer1 , a key miRNA processing enzyme, and quantified miR-223 levels by real-time PCR. Dicer1 mRNA levels were found to be decreased ~65% in Dicer siRNA-treated cells; however, we found no difference in cellular miR-223 levels between HCAEC with or without Dicer knockdown ( Fig. 3f ). HDL-associated miRNAs are likely protected from circulating RNases in blood through their association with HDL lipids and proteins [40] . When the RNAse A-treated HDL were incubated with HCAEC, the miR-223 content of the cells was significantly lower than what was observed in the cells that were incubated with untreated HDL ( Supplementary Fig. 7 ). To determine miRNA changes in HDL before and after incubation with HCAEC, we used TaqMan Low-Density miRNA Arrays to quantify these changes. HDL-miR-223 levels were found to be significantly decreased after incubation with HCAEC (−13.64-fold, unpaired t -test P <0.05, n =4, Fig. 3g ). This was further confirmed by individual TaqMan assays ( Fig. 3h ). The lack of miR-223 transcription in HCAEC was further confirmed by mining previously reported data sets from the ENCODE project [41] and analysing the region corresponding to the pri-mir-223 promoter. When compared with GM12878 (lymphoblast) and K562 (myeloblastoid) human cell lines, in which the promoter region of miR-223 has very strong signals for open chromatin (DHS) and active transcription (K4me3, K36me3 and K27ac); at this time no evidence suggests that these signals are apparent in endothelial cells (HUVECs) ( Supplementary Fig. 8 ). HDL-miR-223 represses ICAM-1 expression and function miRNA target prediction software (TargetScan) was used to identify potential miR-223 target genes in endothelial cells. The results established that human ICAM-1 harbours one broadly conserved putative miR-223 target site within its 3′ untranslated region (3′ UTR) ( Supplementary Fig. 9A ). Based on these data, we hypothesized that the anti-inflammatory capacity of HDL is conferred in part by its ability to transfer miR-223 to endothelial cells where it represses ICAM-1 expression. To determine whether miR-223 directly targets ICAM-1 mRNA at this predicted target site, HEK 293 cells were co-transfected with ICAM-1 –3′ UTR luciferase reporters and a miR-223 mimetic. Over-expression of miR-223 significantly reduced normalized (Firefly/ Renilla ) luciferase activity in HEK 293 (Mann–Whitney nonparametric test P <0.01, Fig. 4a ). To determine whether the predicted miR-223 target site is functional, HEK 293 cells were also co-transfected with miR-223 and an ICAM-1–3′ UTR reporter construct containing a three-base deletion in the middle of the predicted miR-223 seed site (3′ UTR 814–816). The target site three-base deletion abolished the capacity of miR-223 to inhibit ICAM-1 –3′ UTR luciferase activity. To demonstrate that HDL deliver functional miR-223 that directly targets and represses ICAM-1 gene expression, HCAEC were electroporated with luciferase gene reporters containing the full-length ICAM-1 –3′ UTR. We found significant loss of normalized (Firefly/ Renilla ) luciferase activity after HCAEC were incubated with native HDL (1 mg protein per ml) ( Fig. 4b , Mann–Whitney non-parametric test P <0.01). Moreover, native HDL failed to reduce luciferase activity in HCAEC that were electroporated with mutant reporters where the putative miR-223 target site was disrupted with the three-base deletion. These findings strongly suggest that HDL repression of ICAM-1 is mediated, at least in part by miR-223 directly targeting the 3′ UTR of ICAM-1 in HCAEC. Figure 4: miR-223 directly target ICAM-1 in HCAEC. ( a ) Normalized (Firefly/ Renilla ) luciferase activity in HEK 293 cells dual transfected for 48 h with miR-223 and luciferase gene reporters containing the full-length ICAM-1–3′ UTR, a three-nucleotide (814–816) deletion in the predicted miR-223 target site or a control-3′ UTR. N =3–9 ( b ) Normalized (Firefly/ Renilla ) luciferase activity in HCAEC transfected with luciferase gene reporters containing the full-length ICAM-1–3′ UTR, a three-nucleotide (814–816) deletion or control-3′ UTR for 24 h and incubated for a further 24 h with or without native HDL. N =3–18 ( c ) ICAM-1 mRNA levels in HCAEC transfected (48 h) with miR-223, control siRNA or targeting pool siRNA ICAM-1. N =5–7 ( d ) ICAM-1 protein levels 24, 48 and 72 after HCAEC were transfected with miR-223, ICAM-1 siRNA or control siRNA, as quantified by flow cytometry. N =4 ( e ) ICAM-1 protein levels in HCAEC 72 h after miR-223, control siRNA or ICAM-1 siRNA transfection followed by ±TNF-α (2 ng ml −1 ) for 5 h. N =3–4 ( f ) ICAM-1 protein levels in HCAEC transfected with miR-223 hairpin inhibitor, or ICAM-1 siRNA for 24 h followed by native HDL or PBS incubations (16 h) and ±TNF-α for a further 5 h. N =3–6 ( a – f ) All data are represented as mean±s.e.m. ( g , h ) Neutrophil-binding assays in activated HCAEC as described in the Supplementary Information N =4. The numbers of adherent neutrophils are presented with values representing the mean+s.e.m. Unpaired two-tailed Student’s t -test was used when comparing two groups with a sample size ≤3. Mann–Whitney nonparametric test was used to compare two independent groups with a sample size >3. When data were paired and samples size was >3, Wilcoxon matched-pairs tests were used. To compare three or more unmatched groups, one-way ANOVA and Tukey’s multiple comparisons post-test were used. * P <0.05, ** P <0.01. Full size image To determine whether ICAM-1 mRNA and protein levels are reduced when cellular miR-223 levels are increased, HCAEC were transiently transfected with miR-223 mimics, and ICAM-1 mRNA levels were found to be significantly decreased ( Fig. 4c ). Likewise, ICAM-1 protein levels were also found to be significantly decreased, as assessed by western blotting ( Supplementary Fig. 9B ) and flow cytometry ( Fig. 4d ). Transfection of HCAEC with miR-223 mimics also inhibited the ability of TNF-α to increase endothelial cell ICAM-1 expression ( Fig. 4e ). To demonstrate that HDL repression of ICAM-1 is dependent upon miR-223 transfer and activity, we quantified HDL repression of ICAM-1 protein expression in HCAEC in which miR-223 activity was inhibited using a miR-223-specific hairpin inhibitor. Strikingly, we found that HDL were no longer able to decrease endothelial cell ICAM-1 expression in both non-activated and TNF-α-activated cells ( Fig. 4f , Supplementary Fig. 10 ). ICAM-1 siRNA was used as a control ( Fig. 4c–f ). As previously reported [42] , HDL treatments were found to significantly inhibit neutrophil binding to activated HCAEC (one-way ANOVA and the Tukey’s multiple comparisons post-test P <0.05, Supplementary Fig. 11 ). To investigate the functional impact of increasing mature miR-223 levels in HCAEC on neutrophil adhesion, binding assays were carried out in TNF-α-activated HCAEC. We found that neutrophil adhesion was inhibited equally effectively by HDL and miR-223 (one-way ANOVA and the Tukey’s multiple comparisons post-test P <0.05, Fig. 4g,h ). To additionally demonstrate that the transfer of miR-223 from HDL to HCAEC represses inflammatory gene expression, HCAEC were treated with HDL from wild-type (WT) or miR-223 −/− mice. First, we compared miR-223 levels on mouse and human HDL isolated by fast-protein liquid chromatography (FPLC) and found that mouse HDL has less miR-223 than human HDL ( Fig. 5a ), and we found the presence of miR-223 in HDL from WT mice, but not miR-223 −/− mice. Most interestingly, intracellular levels of miR-223 were significantly less in HCAEC treated with HDL from miR-223 −/− compared with WT HDL ( Fig. 5b ). Strikingly, mRNA levels for two inflammatory genes, ICAM-1 and CSF2 , were found to be significantly increased in HCAEC treated with HDL from miR-223 −/− mice compared with WT mice ( Fig. 5c ). Similar to ICAM-1, CSF2 is also a predicted target of miR-223 ( Fig. 5d ). Figure 5: HDL repression of inflammatory gene expression in HCAEC. ( a ) RQV of miR-223 levels in HDL isolated from human and mouse plasma by fast-protein liquid chromatography (FPLC). Mouse plasma was pooled from six miR-223 −/− mice and 12 WT mice for FPLC separation. ( b , c ) HCAEC were incubated with pooled native HDL (final total protein concentration 1 mg ml −1 ) from WT or miR-223 −/− mice for 24 h. ( b ) miR-223 levels were quantified by real-time PCR and normalized to U6 levels (RQV=2 −(miR-223 Ct—U6 Ct) ). ( N =2–3). ( c ) ICAM-1 and CSF2 mRNA levels were quantified by real-time PCR and normalized to peptidylprolyl isomerase A (PPIA) levels (RQV). ( N =2–3). ( d ) Predicted miR-223 target site within the 3′ untranslated region (3′ UTR) of the CSF2 (mRNA) gene. Full size image Both HDL and miRNAs have been reported to regulate many key processes in endothelial cells, including angiogenesis, senescence, differentiation and inflammation [7] , [12] , [21] , [43] , [44] , [45] , [46] . In the present study, we found that HDL and their lipid and apolipoprotein constituents each induce distinct gene changes and post-transcriptional regulation. Indeed, significant up- and downregulation of specific endothelial miRNAs were observed after HDL, lipid-free apoA-I, rHDL and SUV treatments. Here we demonstrate that miR-223 is transferred from native HDL to endothelial cells, miR-223 is not transcribed in HCAEC and HDL do not induce miR-223 transcription in endothelial cells, and miR-223 directly targets ICAM-1 in HCAEC. These data support that HDL-miR-223 delivery confers, in part, HDL’s anti-inflammatory capacity in endothelial cells. Native HDL is composed of many constituents, including bioactive lipids, apolipoproteins, other proteins and miRNAs [14] , [47] , [48] . The extent to which these constituents contribute to HDL-mediated gene regulation has not been systematically examined. One of the key outcomes from this present study is that the individual constituents of HDL each alter the expression of distinct sets of genes in endothelial cells. Many of these genes were significantly altered in the same direction by lipids (SUV), rHDL and native HDL treatments; and were thus classified as the ‘cholesterol efflux responsive gene set’, as the common feature of each condition is the capacity to accept free cholesterol. The ‘cholesterol efflux responsive gene set’ in HCAEC significantly modulate distinct pathways including interferon signalling, LXR/RXR activation and other inflammatory pathways (p38 MAPK signalling, IL22 signalling, role of JAK1, JAK2 and TYK2 in interferon signalling, role of JAK family kinases in IL-6-type cytokine signalling). It is noteworthy that HDL also inhibit the expression of similar inflammatory pathways in macrophages by activating signalling cascades through ABCA1 (refs 49 , 50 ), which was associated with membrane cholesterol levels [51] , [52] . Indeed, multiple studies have found that HDL alter gene expression in cells that they interact with, including macrophages [49] . The present study shows that HDL treatment in endothelial cells resulted in the differential expression of multiple STAT3 target genes in HCAEC, including nine genes recently identified as STAT3 target genes [53] . Most interesting, ABCA1, the expression of which was significantly decreased in HCAEC incubated with HDL in the present study, was also found to be a STAT3 target gene. HDL suppression of ABCA1 was an unexpected finding and may be part of a novel feedback mechanism to counter cellular cholesterol efflux; however, this will require further investigation. Likewise, it is currently unknown whether this suppression is mediated through post-transcriptional regulation, possibly through HDL-induced miRNA changes, or through inhibition of transcriptional activation through any number of transcription factors, including liver x receptors (LXR) or Sp1 (refs 54 , 55 , 56 ). Pathway analysis of gene expression indicated that the NF-κB signalling pathway in HCAEC was significantly decreased by HDL. This is consistent with earlier studies in which HDL inhibited TNF-α-induced adhesion molecule as well as cytokine and chemokine expression in HCAEC and HUVEC [7] , [57] . Here we report that HDL markedly repressed ICAM-1 and VCAM-1 expression in non-activated HCAEC. These results suggest that HDL inhibit endothelial cell activation likely in part of a homoeostatic gene regulatory network. The ability of HDL to inhibit inflammation in endothelial cells in the current study is not limited to adhesion molecule expression, with many cytokines and chemokines, including CCL20, CXCL1 and CSF2, being downregulated. In addition, PRDM1, a transcriptional repressor and master regulator of antibody-producing cell maturation [39] and interferon signalling, were also found to be significantly inhibited by HDL treatments ( Supplementary Table 3 ). The physiological relevance of this control remains to be determined; however, HDL control of transcription factor activities, namely PRDM1, will be of significant interest in future studies. In 2011, we reported that HDL transport specific miRNAs [14] and miR-223 was found to be the most significantly upregulated miRNA in HDL from human subjects with familial hypercholesterolaemia, an inheritable disorder associated with markedly elevated plasma cholesterol levels, premature atherosclerosis and vascular inflammation [14] . miR-223 has been reported to be a myeloid-specific miRNA and is highly expressed in neutrophils and macrophages [29] ; mature miR-223 is also present in other non-myeloid cell types, including endothelial cells [27] , [58] . In our previous study, we reported that macrophages export miR-223 to HDL and that HDL delivers miR-223 to Huh7 hepatoma cells where it regulates gene expression [14] . In this study, we report that HDL and their constituents each regulate distinct miRNAs in endothelial cells. Nevertheless, HDL-induced miR-223 upregulation was unique to native HDL. Therefore, we hypothesized that miR-223, one of the most abundant miRNAs on native human and mouse HDL [14] , was transferred from HDL to endothelial cells where it directly regulates target gene expression, including ICAM-1, which harbours a strong predicted miR-223 target site that is broadly conserved amongst vertebrates. In this study, we establish that mature miR-223 is abundant in endothelial cells (HCAEC and HUVEC) where it is neither transcribed nor processed. This is explained by the transfer of mature miR-223 from HDL to both HCAEC and HUVEC. The present report extends this finding by establishing that HDL also transfers functional miR-223 to HCAEC where it controls inflammatory gene expression. It is therefore likely that, in the context of atherosclerosis and other inflammatory diseases, macrophages export miR-223 to HDL, which in turn transfer miR-223 to endothelial cells as a feedback mechanism to antagonize inflammation. The levels of extracellular miRNAs, specifically HDL-miR-223 levels, are altered in disease states, including atherosclerosis and cardiovascular disease [14] , [21] . The functional impact of HDL-associated miR-223 in the development and resolution of atherosclerosis remains to be determined; however, results from this study support a role in vascular inflammation. Although little is currently understood concerning the functional relevance of extracellular miRNAs in vivo , multiple studies in vitro clearly support that extracellular miRNAs are likely transferred to recipient cells. We have previously reported that HDL-miRNAs are taken up by HDL’s receptor, scavenger receptor BI (SR-BI), in Huh7 cells and in SR-BI-overexpressing baby hamster kidney cells [14] . Endothelial cells also express SR-BI and we predict that HDL-miRNA transfer to HCAEC is also mediated through SR-BI. However, endothelial cells also express other scavenger receptors that have been found to take up HDL-cholesteryl esters, including CD36 (refs 59 , 60 ). Currently, it is unclear whether other HDL receptors take up HDL-miRNAs and whether other delivery mechanisms transfer functional miRNAs to the cytoplasm of recipient cells. Likewise, it is unknown whether HDL–miRNA intercellular communication is limited to only SR-BI-expressing cells. Future studies will be required to demonstrate the functional role of SR-BI in HDL-miRNA communication in vivo . Furthermore, it is unknown how HDL-transferred miRNAs escape the plasma membrane and whether they are loaded onto endogenous RNA-induced silencing complexes (RISC) and target mRNAs through canonical post-transcriptional mechanisms or whether they utilize other cellular machinery and mechanisms to recognize and translationally repress targeted mRNAs. Argonaute 2 ( AGO2 ), the structure–function protein of RISC, is predicted to prefer double-stranded duplexed miRNAs; however, HDL-miRNAs are likely single-stranded and may be differentially loaded onto AGO2-RISC or other AGO family members. If extracellular miRNAs regulate gene expression though distinct mechanisms from endogenous miRNAs, cellular gene regulation may include bias and differential sensitivity to either class. Moreover, HDL-miRNA delivery through SR-BI may bypass endosomal transport and lysosomes that may degrade extracellular RNAs, unlike receptor-mediated endocytotic mechanisms. As such, differential modes of uptake likely are associated with varied functional integrity of the extracellular miRNAs in recipient cells. In summary, we present evidence that HDL and their individual constituents differentially alter miRNA and gene (mRNA) profiles in endothelial cells. We also report that native HDL transfer mature miR-223 to endothelial cells and miR-223 downregulates ICAM-1 expression. To our knowledge this is the first report of the presence of a mature miRNA actively controlling gene expression in a cell in which it was not transcribed or processed. These results not only confirm that miR-223 functions as a suppressor of inflammation in activated and non-activated endothelial cells but also provides a novel insight into the mechanism of the anti-inflammatory properties of HDL. Isolation and characterization of native HDL and lipid-poor apoA-I Blood was collected from five normal healthy donors (three females and two males, aged 25–35 years old) into EDTA-Na 2 tubes and from autologously donated, pooled blood samples from normal healthy donors (Healthscope Pathology, Australia). Native high-density lipoproteins (HDL) were isolated by sequential ultracentrifugation in the 1.063<d<1.25 g ml −1 density range [61] , and the HDL isolated from the autologously donated blood were delipidated using standard techniques [62] . Briefly, 10 ml methanol was added to 1–2 ml of partly lyophilized HDL and the mixture was vortexed and left at room temperature for 1–3 h or until the precipitate was clearly visible. Chloroform (10 ml) was added and the solution was vortexed and left at room temperature for 10–30 min. Chilled ether (33 ml) was then added and the mixture was chilled for 30 min. The mixture was then spun (1,500 r.p.m., 4 °C) for 10 min and the supernatant was removed. Methanol (10 ml) was added to the pellet and the mixture was briefly vortexed. Chilled ether (43 ml) was added to the mixture, which was chilled for an extra 15 min. The mixture was spun (1,500 r.p.m., 4 °C) for 10 min and the supernatant was removed. Methanol (10 ml) was again added to the pellet and the chilled ether wash was performed twice. The resulting pellet was dried using nitrogen then dissolved in 2 ml of 20 mM Tris (pH 8.2). Apolipoprotein (apo) A-I was isolated from the resulting apoHDL by anion exchange chromatography [63] on a Q Sepharose Fast Flow column attached to an FPLC (Äkta) system (GE Healthcare, Chalfont St Giles, Bucks, UK). As judged by electrophoresis on a homogeneous 20% SDS-Phast gel (GE Healthcare Bio-Sciences) and Coomassie staining, the apoA-I was >95% pure. Informed consent was obtained from all subjects and the human research ethics committee (University of New South Wales) approved these studies. Plasma concentration of human HDL constituents Blood was collected from five normal healthy donors (same as above) into EDTA-Na 2 tubes and native HDL were isolated using the Polyethylene Glycol 6000 (PEG-6000) method [64] . Briefly, 1:1 v / v ratio of plasma and PEG were mixed. LDL/VLDL were allowed to precipitate for 20 min on ice. The mix was centrifuged (15,000 r.p.m., 20 min) to pellet the LDL/VLDL fraction. The supernatant (HDL fraction) was carefully removed using a pipette. The plasma concentration of the human HDL constituents, including apolipoprotein A-I (apoA-I), apolipoprotein A-II (apoA-II), total cholesterol (TC), unesterified cholesterol (UC); cholesterol esters (CE=TC-UC) and triglyceride (TG) were determined enzymatically on a Beckman Coulter AU480 Auto-Analyser (Beckman Coulter, Inc.; CA, USA). Preparation and characterization of discoidal reconstituted HDL (rHDL) rHDL containing apoA-I and 1-palmitoyl-2-linoleoyl phosphatidylcholine (PLPC; Avanti Polar Lipids, Alabaster, AL) (initial PLPC:apoA-I molar ratio 100:1, final PLPC:apoA-I molar ratio 80:1) were prepared by the cholate dialysis method [65] . Briefly, 53.06 μl of PLPC (100 mg ml −1 ) was dried as a thin layer in a glass tube using nitrogen. Sodium cholate (100.47 μl; 30 mg ml −1 ) was added and the tubes were briefly mixed. TBS was added to give a final volume of 500 μl. The mix was vortexed every 15 min and allowed to stand on ice until the mixture was optically clear. ApoA-I (2 mg) was added and the mixture was allowed to stand on ice for an extra 2 h. The pooled mixtures were then dialysed (five times) against 1 l TBS over 5 days. Particle sizes were determined by electrophoresis on 3–40% non-denaturing polyacrylamide gradient gels and Coomassie staining with reference to high-molecular weight standards of known diameter [66] . Preparation of SUV PLPC SUV were prepared as described [67] . Briefly, PLPC (39 μl of a 100 mg ml −1 solution in ChCl 3 /MeOH (2/1, v / v )) was mixed with 20 μl of 1 mM butylated hydroxytoluene (BHT). The mixture was dried under a rapid stream of nitrogen for 2 h at 40 °C. PBS was added to the dried lipids and the mixture was sonicated for 5 min bursts in an ice bath until optically clear. The solution was centrifuged for 10 min at 15,000 r.p.m. and the supernatant (SUV) was collected. The phospholipid concentration was determined enzymatically on a Roche Diagnostic/Hitachi 902 Auto-Analyser (Roche Diagnostics GmbH, Mannheim Germany) [68] . Cell culture HCAEC and HUVEC (Cell Applications, Inc. San Diego, CA), passages 3–6, were grown in MesoEndo Growth Medium (Cell Applications, Inc.) containing 5% ( v / v ) serum and plated 24 h before use in 12 well plates at a density of 1 × 10 5 cells per well. HCAEC were incubated at 37 °C for 16–24 h with SUV (final PLPC concentration 3 mmol l −1 ), lipid-free apoA-I (final concentration 1 mg ml −1 ), rHDL (final apoA-I concentration 1 mg ml −1 ), native HDL (final total protein concentration 1 mg ml −1 ) or PBS. To determine whether HDL transport and deliver miR-223 to HCAEC, we examined HDL-associated miRNA profiles before and after 16 h of incubation with HCAEC using real-time PCR-based TaqMan miRNA arrays. Results were validated with individual TaqMan miRNA assays. To determine whether HDL induce miR-223 transcription, HCAEC were treated with native HDL particles in the presence of Actinomycin D (5 μg ml −1 ). HCAEC were also transfected with miR-223 mimetics (100 nM). mRNA and protein levels of ICAM-1 were assessed using real-time PCR, western blotting and flow cytometry. Whole-genome microarrays HCAEC were incubated at 37 °C for 16 h in a 5% ( v / v ) lipoprotein-depleted serum medium with either native HDL from each of five donors (final protein concentration 1 mg ml −1 ), rHDL (final apoA-I concentration 1 mg ml −1 ), lipid-free apoA-I (final concentration 1 mg ml −1 ), SUV (final PLPC concentration 3 mmol l −1 ) or PBS. The cells were harvested and total RNA was isolated using Qiazol miRNAeasy kits (Qiagen) and quantified by spectrophotometry (Nanovue). Gene expression profiling was assessed using Affymetrix GeneChip microarray assays according to the manufacturer’s protocol (Affymetrix). Briefly, 1 μg of total RNA was reverse transcribed (T-7 dT primers), amplified and biotinylated (Affymetrix IVT Labelling Kit). Samples were hybridized to GeneChip Human Gene 1.0 ST whole-genome arrays (28,869 genes) (Affymetrix), washed, stained (Affymetrix Fluidics Station) and scanned (Affymetrix GeneChip Scanner). Relative quantitative values (RQV) were used to determine mRNA levels; RQV=2 −d C t . microRNA microarrays HCAEC were incubated at 37 °C for 16 h in a 5% ( v / v ) lipoprotein-depleted serum medium with either native HDL from each of five donors (final protein concentration 1 mg ml −1 ), rHDL (final apoA-I concentration 1 mg ml −1 ), lipid-free apoA-I (final concentration 1 mg ml −1 ), SUV (final PLPC concentration 3 mmol l −1 ) or PBS. Cells were harvested for real-time PCR TaqMan miRNA arrays (see below). Native HDL were extracted from the medium by immunoprecipitation using 400 μl of 5.2 mg ml −1 goat anti-human apoA-I microbeads (Academy Bio-Medical Company, Houston, TX, USA). HDL-miRNA profiles before and after incubation with HCAEC were assessed by real-time PCR TaqMan miRNA arrays (see below). Total RNA was isolated from HCAEC and native HDL pre- and post-incubation with HCAEC by Qiazol miRNAeasy kits (Qiagen) according to the protocol described by the manufacturer. Reverse transcription was performed using Human MegaPlex RT Primer pools. cDNA was amplified using human MegaPlex PreAmp Primer Pools and PreAmp Master mix. The amplified samples were loaded into Taqman microRNA arrays (Part Number 4444913) Pool A (377 miRNAs) and pool B (373 miRNAs) and analysed using the 7900 Real Time PCR System (Applied Biosystems). C t values were calculated by SDS 1.2 software (Applied Biosystems) and normalized to MammU6 (miRNA) housekeeping C t values and expressed as 2 −( C t(microRNA)−Ct(U6)) . For the miRNA isolated from HDL pre- and post-incubation with HCAEC, results (Cts) were normalized to the HDL total protein concentration determined by the BCA assay (Thermo Scientific, USA). Primary miRNA, precursor miRNA and mature miRNA individual TaqMan Assays Total RNA was purified as outlined above and reversed transcribed using the TaqMan microRNA reverse transcription kit (Applied Biosystems) according to the manufacturer’s protocol. Subsequently, the reverse transcription product was used for detecting miRNA expression by real-time PCR using individual TaqMan miRNA Assay Kits (Applied Biosystems) for the specific miRNAs ( Supplementary Table 8 ). Values were normalized to U6 and expressed as 2 −( C t(microRNA)− C t(U6)) . For the quantification of pri-miRNA, total RNA (900 ng) was reversed transcribed using the High capacity RNA-to-cDNA kit (Applied Biosystems) according to the instructions of the manufacturer. The reverse transcription product (1.5 μl) was used for detecting pri-miRNA expression by qPCR using TaqMan Pri-miRNA Assays (Applied Biosystems) for specific pri-miRNA ( Supplementary Table 8 ). Real-time PCR was performed with MyiQ single colour real-time PCR detection system, using iQ SYBR Green Supermix (Bio-Rad) for relative mRNA quantification of precursor miR-223. Values were normalized to human actin and expressed as 2 −( C t(Pri-microRNA]− C t(Actin)) or normalizing Cts to PPIA. See Supplementary Table 8 for details. Transfections of HCAEC HCAEC were plated at a density of 1 × 10 5 per well 24 h prior to transfection. Transient transfections (50–100 nM, DharmaFECT 4, Dharmacon) were conducted for 48 h with hsa-miR-223 miRIDIAN mimic, human Dicer (ON-TARGETplus SMARTpool Dharmacon), miR-223 hairpin inhibitors (100 nM) or siRNA against human ICAM-1 (ON-TARGETplus SMARTpool Dharmacon). siRNAs Dharmacon catalogue numbers are listed in Supplementary Table 8 . Real-time PCR Total RNA was isolated from HCAEC using miRNeasy mini kit (Qiagen) or Total RNA Purification kits (Norgen). Reverse transcription was performed using 0.1 μg of RNA. Real-time PCR was performed with MyiQ single-colour real-time PCR detection system, using iQ SYBR Green Supermix (Bio-Rad) for relative mRNA quantification. Specific mRNAs were also quantified by specific TaqMan probes (Life Technologies). PCR primers and TaqMan Probes are listed in Supplementary Table 8 . Western blots Cells were washed with ice cold PBS and lysed in 20 mM Tris buffer (pH 7.5), containing 0.5 mM EDTA-Na 2 , 0.5 mM EGTA-Na 2 and proteases inhibitors. Cellular proteins were resolved by SDS–PAGE and transferred electrophoretically to nitrocellulose membranes. The membranes were incubated overnight using mouse anti-human monoclonal antibodies directed against ICAM-1 (1:500) and β-actin (1:3,000) (Abcam, Cambridge, UK, all). Respectively, 1:500 and 1:5,000 dilution anti-mouse IgG-HRP (Abcam) were used as secondary antibodies. Immunoreactive proteins were detected by chemiluminescence and analysed using Quantity One 1-D Analysis Software (Bio-Rad). Flow cytometry Cell surface ICAM-1 expression in HCAEC was determined by flow cytometry (Beckman Coulter FC500, Fullerton, CA, USA) using FITC-ICAM-1 fluorescent antibodies. A FITC IgG1 isotype non-specific antibody was used as negative control (BD Pharmingen). Briefly, adherent cells were washed with cold PBS and then incubated for 30 min at 4 °C with 250 μl of either ICAM-1 antibody or IgG1 isotype non-specific antibody (PBS+10% human serum). Cells were washed with cold PBS then detached using 2 mM EDTA in PBS. EDTA was neutralized with PBS containing 10% human serum. Cells were transferred to eppendorf tubes and washed (2–3 times) with PBS. Cell pellets were re-suspended in PBS containing 2% human serum. Flow cytometry analyses were performed and forward scatter versus side-scatter gates were set to include only viable cells. A number of events between 5,000 and 10,000 cells was analysed for each sample with a minimum of 65% viable cells. Changes in mean fluorescence intensity were recorded. 3′ UTR luciferase reporter assays HEK 293 and HCAEC were transfected for 48 h with 500 ng of the complete ICAM-1 3′ UTR (ICAM-1 1,331 bp, product ID: HmiT009184) hLuc-hRLuc luciferase reporter vector (GebeCopoeia, Rockville, MD, USA) or 500 ng of the control construct (ENHO—Energy Homoeostasis). HEK 293 cells were co-transfected with or without 100 nM of hsa-miR-223 miRIDIAN mimic. HCAEC were incubated with or without HDL (1 mg total protein per ml) 24 h before harvesting the cells. HEK 293 cells were transfected using DharmaFECT 4 transfection reagent (Dharmacon). HCAEC were transfected by electroporation using the Neon Transfection kit and device (Life Technologies, NY, USA). The cells were washed with PBS and lysed using Cell Culture Lysis Reagent (Promega, Madison, WI, USA). Luciferase activities (luminescence ratio of Firefly /Renilla ) were measured using the Luc-Pair miR Luciferase Assay Kit (GebeCopoeia, Rockville, MD, USA). Site-directed mutagenesis Three bases (814–816) in the ICAM-1 3′ UTR plasmid construct were deleted using the QuickChange II XL Site-Directed mutagenesis Kit (Agilent Technologies). Briefly, the QuikChange II XL site-directed mutagenesis method was performed using PfuUltra high-fidelity (HF) DNA polymerase for mutagenic primer-directed replication of both plasmid strands. The oligonucleotide primers, each complementary to opposite strands of the vector, were extended during temperature cycling by PfuUltra HF DNA polymerase, without primer displacement. Forward 5′-ATTCCTCCCTTCCCCCCA AAAACACCTTTGTTAGC-3′ and reverse 5′-GCTAACAAAGGTGTTTTTGGG GGGAAGGGAGGAAT-3′ primers were used at a concentration of 125 ng μl −1 . Extension of the oligonucleotide primers generated a mutated plasmid containing staggered nicks. Following temperature cycling, the product was treated with Dpn I. The Dpn I endonuclease (target sequence: 5′-Gm6ATC-3′) is specific for methylated and hemi-methylated DNA and was used to digest the parental DNA template and to select for DNA containing the deletion. DNA isolated from almost all E. coli strains is dam-methylated and therefore susceptible to Dpn I digestion. The nicked vector DNA incorporating the desired deletions was then transformed into XL10-Gold ultracompetent cells. HEK 293 cells and HCAEC were transfected with the mutated ICAM-1 3′ UTR hLuc-hRLuc luciferase reporter vector (500 ng) with or without 100 nM of hsa-miR-223 for HEK 293 cells and with or without HDL for HCAEC (described above). The three-base deletion was confirmed by sequencing. Neutrophil-endothelial cell attachment assay HCAEC were grown in MesoEndo medium containing 5% ( v / v ) serum and plated on glass coverslips in 12 well plates at a density of 1 × 10 5 cells per well. Cells were transiently transfected for 48 h before use with 100 nM hsa-miR-223 miRIDIAN mimic or siRNA control using the method described above. Native human HDL (final protein concentration 1 mg ml −1 ) or PBS was added 16 h before use. After 48 h of transfection, cells were then incubated at 37 °C for 5 h in the presence or absence of TNF-α (2 ng ml −1 ). Human neutrophils were isolated using Polymorphprep (Axis-Shield, Olso, Norway) and incubated for 15 min at 37 °C with 25 μM of the cell-tracing reagent, CellTrace CFCE cell proliferation kit (Molecular Probes, Inc. Eugene, OR). Fluorescently labelled, isolated human neutrophils (1 × 10 6 , 100 μl) were added to HCAEC and incubated for 2 h. The cells were gently washed with PBS (3 × ) and fixed on a slide using mounting media (Vectashield, Vector Laboratories Inc., Burmingame, CA, US). Fluorescently labelled cells were visualized on an inverted microscope and the number of adherent neutrophils was counted using Image J software (NIH, US) [42] . Results are shown with values representing the mean ±s.e.m. RNAse A digestion Density-gradient-ultracentrifuged purified native HDL was digested with RNAse A (400 μg per mg total HDL protein) at 37 °C for 2 h followed by the addition of 2 × RNAse inhibitor for 30 min at 37 °C to stop reaction. Treated and control (no RNAse A) HDL were incubated with HCAEC for 24 h at a final concentration of 1 mg ml −1 . Treated cells were extensively washed and total RNA was isolated for downstream transcriptomics. miR-223 −/− mouse experiments HDL was isolated from adult (2–6 months) miR-223 −/− or C57BL/6 wild-type (WT) mouse plasma using fast-protein liquid chromatography (FPLC). HCAEC were treated for 24 h with pooled native HDL (final total protein concentration 1 mg ml −1 ) from 12 WT (mixed gender, 6 males and 6 females) mice or 6 miR-223 −/− mice (mixed gender, 5 males and 1 females). Mouse miR-223 (mmu-miR-223) levels in HDL and HCAEC (incubated with HDL) were quantified by real-time PCR and normalized to U6 levels (HCAEC, RQV=2 −(Ct(miR-223)–Ct(U6) ) or arbitrary C t=32 and total HDL protein (HDL). All mouse studies were completed under active National Institutes of Health, National Heart, Lung and Blood Institute Animal Care and Use Committee protocols, and all experiments complied with the criteria outlined in the NIH ‘Guide for the Care and Use of Laboratory Animals’. Informatics miRNA target prediction studies were carried out using TargetScan 5.2. ( www.targetscan.org ). High-level and low-level transcriptomics analyses were carried out using GeneSpring GX12.0 (Agilent) ( www.genomics.agilent.com ). Pathway analyses were carried out with Ingenuity Pathway Analyses. www.ingenuity.com . Statistical analysis Data are presented as mean±s.e.m. When comparing two groups with a sample size ≥3, an unpaired two-tailed Student’s t -test was used. Mann–Whitney nonparametric tests were used to compare two independent groups with a sample size >3. When data were paired and samples size was >3, Wilcoxon matched-pairs tests were used. One-way ANOVA and the Newman–Keuls post-tests were used to compensate for multiple testing procedures. A value of P <0.05 was considered to be significant. How to cite this article: Tabet, F. et al. HDL-transferred microRNA-223 regulates ICAM-1 expression in endothelial cells. Nat. Commun. 5:3292 doi: 10.1038/ncomms4292 (2014). Accession Codes: All array data have been uploaded to Gene Expression Omnibus ( http://www.ncbi.nlm.nih.gov/geo/) under accession codes GSE53201 (HCAEC mRNA Gene Array), GSE53315 (HCAEC miRNA TaqMan low-density array) and GSE53314 (HDL miRNA profiling before and after incubations with HCAEC miRNA TaqMan low-density array).